Entropic cages for trapping DNA near a nanopore Nanopores can probe the structure of biopolymers in solution; however, diffusion makes it difficult to study the same molecule for extended periods. Here we report devices that entropically trap single DNA molecules in a 6.2-femtolitre cage near a solid-state nanopore. We electrophoretically inject DNA molecules into the cage through the nanopore, pause for preset times and then drive the DNA back out through the nanopore. The saturating recapture time and high recapture probability after long pauses, their agreement with a convection–diffusion model and the observation of trapped DNA under fluorescence microscopy all confirm that the cage stably traps DNA. Meanwhile, the cages have 200 nm openings that make them permeable to small molecules, like the restriction endonuclease we use to sequence-specifically cut trapped DNA into fragments whose number and sizes are analysed upon exiting through the nanopore. Entropic cages thus serve as reactors for chemically modifying single DNA molecules. A nanometre-scale pore in a thin membrane can be used to detect a single molecule and sense its physical structure as it passes through the pore while in solution [1] , [2] . Nanopore sensors have enabled fundamental studies on single biopolymers [3] , [4] , [5] , [6] , [7] , [8] , [9] and show promise for use in a variety of biosensing applications [10] , [11] , [12] , [13] , [14] , [15] , [16] , [17] , [18] , [19] . Nanopores are particularly well suited for probing chemical interactions between DNA and other molecules [20] , [21] , [22] , because these interactions often substantially modify the structure of a DNA molecule. For example, oligonucleotide hybridization probes [23] bind to specific DNA target sequences and create bulges that are easy to detect when they pass through a nanopore. Applying this principle, Singer et al . [14] mapped the locations of target sequences on long, double-stranded DNA molecules, and Wanunu et al . [12] identified different microRNAs. To correctly infer that the structure of a DNA molecule has changed, however, it is crucial to know what was the structure of that molecule before the chemical interaction occurred. This presents a serious epistemic challenge, as nanopore sensors should ideally discover the characteristics of a molecule without prior knowledge. A solution is to use a nanopore to characterize the same DNA molecule before and after a chemical interaction; For that, we require what amount to single-molecule test tubes in which DNA can interact with other molecules without diffusing away. Rant et al . [24] took an important step towards that goal when they developed devices comprising two pores and a microscale cavity. They demonstrated that the diffusion of particles and DNA can be significantly slowed inside the cavity [25] . Those devices held DNA molecules in the cavity for only a few seconds, however, which is too short to be practical for studying chemical interactions. (In a separate set of experiments, similar devices were used to measure the transit time of DNA molecules moving between two opposing nanopores by electrophoresis [26] ). Here we report the fabrication and use of devices that juxtapose a solid-state nanopore with a cage that can trap a single DNA molecule for many minutes. The cage is a disc-shaped, micrometre-scale cavity with a few-hundred-nanometre-wide opening in one face and a nanopore in the other. DNA is driven into and out of the cage by electrophoresis through the nanopore. The cage traps DNA entropically [27] , which means that DNA is prevented from diffusing away by the reduction in configurational entropy that would be required for the polymer coil to squeeze through an opening smaller than its radius of gyration [28] . Small molecules like hybridization probes and restriction enzymes can nevertheless diffuse through the opening without difficulty. We experimentally demonstrate that single DNA molecules can be stably trapped in a cage for several minutes and recovered with nearly perfect efficiency. We then demonstrate how our devices can analyse DNA before and after a chemical reaction using a restriction endonuclease to cut DNA held in the cage and detecting the resulting fragments with the nanopore. Entropic cages are useful as single-molecule chemical reactors for nanopore biosensing with a variety of chemical probes [29] , [30] , and for studying biologically significant interactions between DNA and other molecules. 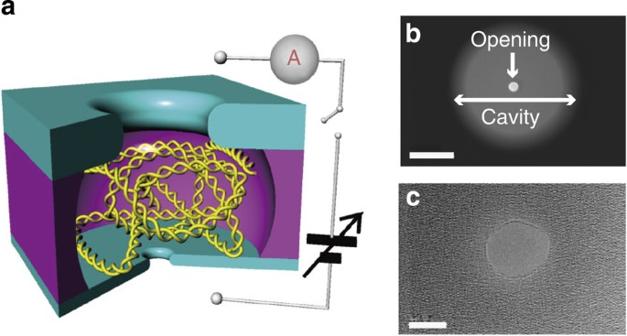Figure 1: The nanopore entropic cage structure. (a) A three-dimensional cutaway illustration of the device. (b) TEM image of the device showing the cavity and the opening. Scale bar, 1 μm. (c) A high-magnification TEM image of the nanopore. Scale bar, 10 nm. Nanopore cage structures and experiments Figure 1a illustrates the nanopore cage structure, and Fig. 1b shows transmission electron microscope (TEM) images of a typical one. The structure is similar to the pore-cavity-pore device developed by Pedone et al . [24] , but it features a cylindrical cavity as opposed to a pyramidal one. Furthermore, we judge our fabrication method to be simpler while granting us better control over the device dimensions. Each structure was made in a freestanding membrane on a silicon chip. The membrane comprised a three-layer stack of materials. The outermost layer, made of low-stress silicon nitride, was 20 nm thick. The middle layer was 1.5 μm thick and made of silicon dioxide. The layer closest to the silicon chip was 400 nm thick and made of low-stress silicon nitride. To create the nanopore cage structures, we first used a focused ion beam machine (FEI Helios) to mill a 200-nm-diameter opening through the innermost layer of silicon nitride. A buffered hydrofluoric acid etch then selectively removed SiO 2 from the middle layer, creating a 1.5-μm-high cavity whose diameter was selected by controlling the duration of the etch. A diameter of 2.3 μm was obtained after 10 min of etching. The cavity was large enough to accomodate a λ DNA molecule, which is 16.5 μm long and has a radius of gyration that is R g =730 nm in equilibrium [31] . Finally, we focused the beam of a TEM (JEOL 2100F) onto the 20-nm-thick silicon nitride layer to mill a ≈10-nm-diameter nanopore through it. Figure 1c shows a TEM image of a nanopore. Table 1 summarizes the dimensions of every device used to generate data presented here. Figure 1: The nanopore entropic cage structure. ( a ) A three-dimensional cutaway illustration of the device. ( b ) TEM image of the device showing the cavity and the opening. Scale bar, 1 μm. ( c ) A high-magnification TEM image of the nanopore. Scale bar, 10 nm. Full size image Table 1 Dimensions of the devices tested and the locations of the corresponding data. Full size table In our DNA-sensing experiments, the chip separated two reservoirs of buffered ionic solution, one contacting the opening of the cavity (the ‘opening side’) and the other contacting the nanopore and containing λ DNA (the ‘nanopore side’). The only fluidic path between the two reservoirs passed through the nanopore, the cavity and the opening. An electrometer biased the opening side to a voltage V relative to the nanopore side and measured the resulting ionic current through the nanopore, I , by means of Ag/AgCl electrodes immersed in the reservoirs. The opening, while small enough to confine λ DNA, was too big to significantly affect the ionic resistance of the device, which was governed by the nanopore. I is the basis of the sensing mechanism: DNA molecules pass through the nanopore due to electrophoresis, and the presence of a molecule inside the nanopore causes a measurable change in I [8] . The time course of I reflects the structure of the molecule [14] , [15] , [22] , [32] . A field-programmable gate array (FPGA) digitized I and enabled real-time control over V in response to changes in I or pre-programmed delays [7] . Dynamics of DNA in entropic cages We investigated the dynamics of λ DNA molecules in the entropic cage with ‘ping–pause–pong’ experiments, illustrated in Fig. 2a . A current trace from a typical experiment is shown in Fig. 2b . The application of V =100 mV resulted in a current of 9.73 nA through the 8.5-nm-diameter nanopore. When a DNA molecule translocated the nanopore into the cage, it caused a transient decrease in I . We call this first translocation signal the ‘ping’. We maintained the positive voltage bias for 2 ms following the ping. The voltage bias was then removed for a pause time, t p , during which the molecule could relax and diffuse within the cavity. We varied t p in experiments between 2 ms and 50 s. Following the pause, we flipped the voltage to V =−100 mV for 5 s. We usually observed another transient conductance drop, which we call the ‘pong’, and attribute to the same DNA molecule returning through the nanopore. The interval of time between the voltage reversal and the pong is t r , the recapture time. In these experiments, the ionic current approached a new open-pore value gradually and reproducibly following a change in voltage, whether or not a molecule had translocated the nanopore. The slow change in the baseline current is therefore related to the instrumentation and the nanopore rather than the DNA [7] . 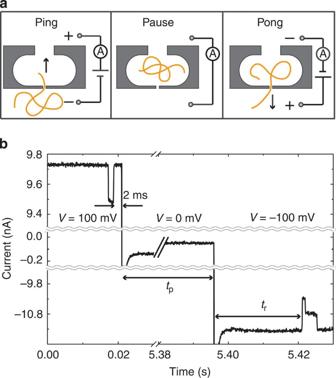Figure 2: Ping–pause–pong experiments. (a) Illustrations of the ping, pause and pong steps of our experiment. (b) A typical current trace from a ping–pause–pong experiment, showing the ping and pong translocation signatures, and illustratingtpandtr. The current transients near 0.02 and 5.39 s were caused by sudden changes inV. The wavy lines indicate breaks in the current axis. Slow drift of the current baseline caused the jump in current observed at the break in the time axis in the pause phase. Figure 2: Ping–pause–pong experiments. ( a ) Illustrations of the ping, pause and pong steps of our experiment. ( b ) A typical current trace from a ping–pause–pong experiment, showing the ping and pong translocation signatures, and illustrating t p and t r . The current transients near 0.02 and 5.39 s were caused by sudden changes in V . The wavy lines indicate breaks in the current axis. Slow drift of the current baseline caused the jump in current observed at the break in the time axis in the pause phase. 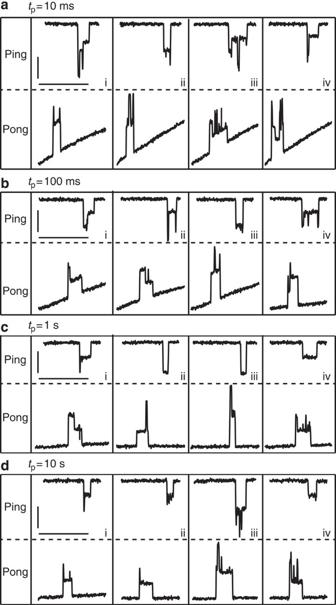Figure 3: Examples of ping and pong translocation events. (a)tp=10 ms, (b)tp=100 ms, (c)tp=1 s and (d)tp=10 s. The paired-event traces are the ping and subsequent pong of the same DNA molecule. All events are plotted on the same scale. The pong event traces fortp=10 ms andtp=100 ms appear on a slanted baseline due to the slow recovery of the baseline current after the voltage change. Horizontal scale bars, 10 ms. Vertical scale bars, 0.2 nA. Full size image Figure 3 shows examples of ping and pong translocation events for delay times ranging from 10 ms to 10 s. Interestingly, the course of the current baseline could be extrapolated continuously across ping and pong events, without any shift resulting from the translocation of a molecule into or out of the cage. The presence of a DNA molecule inside the cage therefore had no observable effect on the access resistance of the device. Figure 3: Examples of ping and pong translocation events. ( a ) t p =10 ms, ( b ) t p =100 ms, ( c ) t p =1 s and ( d ) t p =10 s. The paired-event traces are the ping and subsequent pong of the same DNA molecule. All events are plotted on the same scale. The pong event traces for t p =10 ms and t p =100 ms appear on a slanted baseline due to the slow recovery of the baseline current after the voltage change. Horizontal scale bars, 10 ms. Vertical scale bars, 0.2 nA. Full size image For each DNA translocation, we computed the event charge deficit (ECD), which is the induced current change integrated over the duration of the event. Previous studies showed that ECD is primarily related to the length of a DNA molecule and not the folding configuration in which it translocates [5] , [9] . Since λ DNA is very long, it is an excellent candidate for entropic trapping, but is also relatively easy to break and difficult to purify. Consequently, nanopore studies of λ DNA typically reveal a subpopulation of much shorter molecules [9] , [33] , [34] , [35] (presumably fragments) that could respond differently to an entropic cage, especially if their radius of gyration is smaller than the opening. We have used ECD to identify and remove short fragments of DNA from our data. 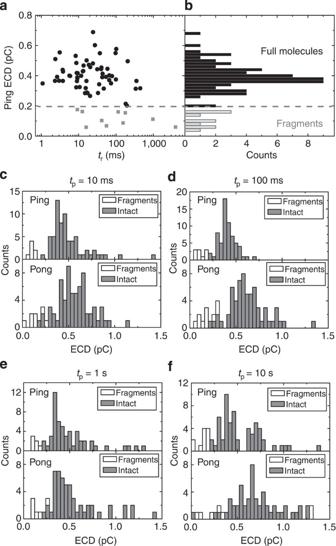Figure 4: Identification and exclusion of DNA fragments. (a) Scatter plot showing the ECD of each ping and the correspondingtrand (b) histogram of the ECD values whentp=30 ms. Data attributed to fragments are shown in grey; these were excluded from subsequent analyses. (c–f) ECD distributions for ping and pong events with (c)tp=10 ms, (d)tp=100 ms, (e)tp=1 s and (f)tp=10 s. Ping events with ECD <0.2 pC are attributed to fragments and indicated by white bars; intact molecules are indicated with grey bars. Figure 4a shows a scatter plot indicating the ECD of each ping and the corresponding t r for t p =30 ms. Most of the data clustered in a major group centred around ECD=0.4 pC and t r =20 ms. A small numer of molecules with low ECD (~0.1 pC) were more broadly distributed in t r , and a few of them exhibited extremely long return times (>1 s). Figure 4b shows the distribution of ping ECD values, which has a major peak near 0.4 pC and a minor tail that is most prominent around 0.1 pC. We attribute the pings in the major group to translocations of intact λ DNA molecules, and those in the minor tail to shorter fragments [9] . We used the threshold ECD=0.2 pC to distinguish between intact molecules and fragments. Figure 4c–f shows ECD distributions from experiments with different t p , while distinguishing between intact molecules and fragments. The distributions of ping ECDs were all similar, showing a main group of translocations that was unaffected by the threshold. Furthermore, molecules identified as fragments based on the ping ECD resulted in low pong ECDs, as expected. Fragments comprised less than 20% of the translocations in every experiment. For the analysis that follows, we only considered the intact molecules. Figure 4: Identification and exclusion of DNA fragments. ( a ) Scatter plot showing the ECD of each ping and the corresponding t r and ( b ) histogram of the ECD values when t p =30 ms. Data attributed to fragments are shown in grey; these were excluded from subsequent analyses. ( c – f ) ECD distributions for ping and pong events with ( c ) t p =10 ms, ( d ) t p =100 ms, ( e ) t p =1 s and ( f ) t p =10 s. Ping events with ECD <0.2 pC are attributed to fragments and indicated by white bars; intact molecules are indicated with grey bars. 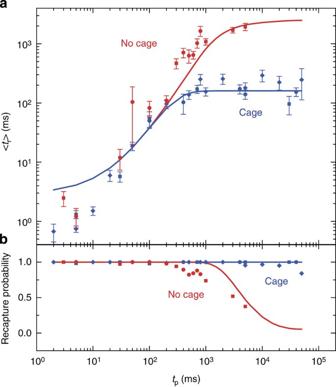Figure 5: Dynamics of DNA in an entropic cage. (a) Dependence of ‹tr› ontpfor devices with an entropic cage (blue) and without (red). Different symbols indicate different devices whose cavity and the opening diameters were, respectively, 2.28 μm and 230 nm (blue squares), 2.25 μm and 230 nm (blue circles), 2.30 μm and 240 nm (blue diamonds), 7.32 μm and 5,320 nm (red squares) and 6.12 μm and 1,560 nm (red circles). The error bars are the s.d. oftr. Seventy ping–pause–pong cycles on average were recorded for eachtp. The solid lines are predictions of the theoretical model described in the text and detailed inSupplementary Note 1. (b) Dependence of the recapture probability ontp. The symbols and lines have the same meanings as ina. The sample sizes inaandbare between 17 and 127, with a mean of 71.3. Full size image Figure 5a shows the dependence of the mean return time ‹ t r › on t p . ‹ t r › increased with t p until t p ≈700 ms, where it saturated at ‹ t r ›≈250 ms (blue data). We determined that the saturation in ‹ t r › was due to the presence of the cage by performing the following control experiments. We applied the same ping–pause–pong procedure, only this time we used a device whose cavity and opening diameters (7.32 and 5.32 μm, respectively) were so much larger than the equilibrium coil size of λ DNA that the cavity could not possibly impede the molecule’s motion. Because of this, the device behaved as if there was no cage at all. The results of these control experiments are shown in Fig. 5a (red squares). ‹ t r › increased with t p over the full range of pause times tested. The longest pause, t p =50 s, gave t r =2 s, which was nearly an order of magnitude longer than the t r plateau value observed in experiments with a cage. Similar results were obtained using a second device with a large 6.12-μm-diameter cavity and a 1.56-μm-diameter opening. Those results are also shown in Fig. 5a (red circles). Figure 5: Dynamics of DNA in an entropic cage. ( a ) Dependence of ‹ t r › on t p for devices with an entropic cage (blue) and without (red). Different symbols indicate different devices whose cavity and the opening diameters were, respectively, 2.28 μm and 230 nm (blue squares), 2.25 μm and 230 nm (blue circles), 2.30 μm and 240 nm (blue diamonds), 7.32 μm and 5,320 nm (red squares) and 6.12 μm and 1,560 nm (red circles). The error bars are the s.d. of t r . Seventy ping–pause–pong cycles on average were recorded for each t p . The solid lines are predictions of the theoretical model described in the text and detailed in Supplementary Note 1 . ( b ) Dependence of the recapture probability on t p . The symbols and lines have the same meanings as in a . The sample sizes in a and b are between 17 and 127, with a mean of 71.3. Full size image The cage also significantly enhanced the probability of recapturing a molecule, defined as the fraction of ping–pause–pong cycles where the ping was followed by a pong. Figure 5b plots the dependence of the recapture probability on t p for translocations into a cage and for translocations across a device with no cage. In the absence of a cage, the recapture probability decreased precipitously with t p for t p >200 ms. The longest pause in the cage-free experiments was 5 s because beyond that, pongs were very rarely detected. By contrast, the recapture probability remained high in devices with a cage, even for t p =50 s (100% for two devices and >80% for a third device). Finally, Fig. 6 plots normalized distributions of 4-μs-long samples of the current blockage caused by translocations, Δ I , for different t p . As has been found previously [36] , translocations produced bimodal distributions of current blockage amplitudes, with a major peak near Δ I =0.13 nA caused by the presence of an unfolded DNA molecule inside the nanopore, and minor peaks at about double the Δ I , corresponding to the presence of a DNA molecule in a folded configuration inside the nanopore. The amplitude of the minor peak relative to the major peak was higher for pongs than for pings, especially for short t p , indicating that folded configurations occurred with greater frequency during the pong. This can be explained by DNA forming a compact coil close to the nanopore immediately after the ping, which increases the frequency of folded configurations during the pong [37] . The peaks in the current blockage distribution of the pongs tended to shift modestly (~10%) towards higher values relative to the pings. We have not determined the reason for this shift. The difference in current blockage distributions was not accompanied by a clear difference in translocation durations between pings and pongs (see Supplementary Fig. 1 ). 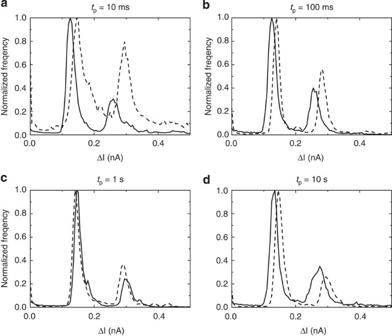Figure 6: Normalized distribution of 4-μs-long samples of the current blockage caused by translocations, ΔI. (a)tp=10 ms, (b)tp=100 ms, (c)tp=1 s and (d)tp=10 s. Solid lines show ping distributions. Dashed lines show pong distributions. Figure 6: Normalized distribution of 4-μs-long samples of the current blockage caused by translocations, Δ I . ( a ) t p =10 ms, ( b ) t p =100 ms, ( c ) t p =1 s and ( d ) t p =10 s. Solid lines show ping distributions. Dashed lines show pong distributions. Full size image Dynamical modelling To guide our interpretations, we modelled the dynamics of DNA in a ping–pause–pong cycle theoretically, and compared the predictions with our experimental results. Our approach was similar to the one used by Gershow and Golovchenko [7] to model the capture and recapture of DNA without a pause step or a cage. We treated λ DNA as a charged particle drifting due to the electric fields outside the nanopore and diffusing at the same time. When a voltage was applied, it induced hemispherically symmetric electric fields that decayed as the inverse square of the distance from the nanopore, as one would expect from a point source of current injected into fluid with a uniform conductivity. Our model used no free parameters; we set the diffusivity of the particle equal to that of λ DNA in a bulk electrolyte [31] , and we took the value of mobility to be μ =2.2 × 10 −4 cm 2 V −1 s −1 in 1 M KCl based on the theoretical estimate by Grosberg [38] . That estimate is consistent with mobility measurements by Stellwagen and Stellwagen [39] if those measurements are extrapolated to a salinity of 1 M . The particle was located 100 nm away from the nanopore at the start of a ping–pause–pong cycle. The evolution of its probability distribution was obtained by numerically solving the convection–diffusion equation in spherical coordinates in the ping and pause phases. To model a DNA trapped in the cage, we imposed an additional, no-flux boundary condition at a radial distance of 1.5 μm away from the nanopore. The pause phase leaves the probability distribution finite at the boundary of the nanopore. If the pong phase was modelled with the convection–diffusion equation by making the nanopore a sink for particles, the probability distribution would be discontinuous there, leading to a singular recapture rate. This creates a computational problem that does not occur in the absence of a pause [7] . We circumvented this problem by ignoring diffusion in the pong phase and instead computing the deterministic drift times of particles back to the nanopore. (See Supplementary Note 1 and Supplementary Fig. 2 for details of this theoretical modelling.) Figure 5a,b shows that the theoretical model is in excellent agreement with the experimental results. Without a cage, ‹ t r › increased monotonically with t p because DNA could diffuse away from the nanopore without bound. The saturation in ‹ t r › obtained from devices with a cage is a clear signature of DNA becoming trapped and returning to the nanopore from a short distance within the cage. The model also provides two explanations for the missing pongs in the experiments with no cage. First, a molecule can diffuse far from the nanopore into the diffusion-dominated region where the electrophoretic force is too weak to drive the molecule back to the nanopore [7] , [38] . Second, it is likely that in some cases we did not wait long enough for the molecule to return to the nanopore. This also explains why ‹ t r › rises slowly with t p after long pauses in experiments with no cage, as these missing pongs would have shown a longer t r than 5 s and they occur more frequently with increasing t p . The model disagrees most with the experimental results in relative terms at short pause times, where t r is predicted to be longer than observed. This error likely stems from treating DNA as a point particle. Since a DNA molecule remains close to the nanopore when t p is short, the distance from the nanopore to the nearest DNA segment can be significantly smaller than the distance to the molecular centre of mass. Therefore, the molecule should be recaptured well before its centre of mass arrives at the nanopore. Visualizing an entropically trapped DNA molecule We visually confirmed that the entropic cage stably trapped λ DNA in a seperate series of experiments. We applied a voltage to pull a DNA molecule into an entropic cage and left it trapped there. We then transferred that chip to an optical microscope, with the opening side facing up, and placed a drop of solution containing the fluorescent dye YOYO-1 onto the chip, as illustrated in Fig. 7a . The YOYO-1 could diffuse through the opening of the cage and stain the DNA molecule inside while we observed the process optically. We located the cavity in white-light mode ( Fig. 7b ) and then monitored that region in flourescence mode for about 25 min, recording an image every 10 s. A bright spot appeared in the location of the cavity ( Fig. 7c ), showing that a DNA molecule was trapped inside. This experiment was repeated on two more nanopore devices and the same result was obtained. 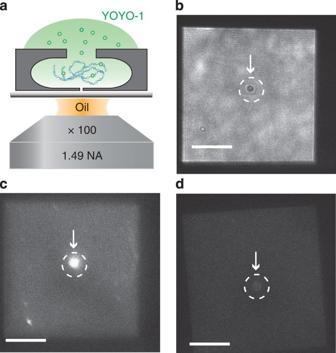Figure 7: Imaging a trapped DNA molecule. (a) Schematic showing one drop of solution containing YOYO-1 fluorescent dye added to the opening side of a chip on an optical microscope. (b) An image of a device with a trapped DNA molecule illuminated by white light. The bright square is the three-layer membrane. The disk indicated by a white dashed circle is the cavity. (c) A fluorescence image of the same device as inb. (d) A fluorescence image of a cage that was emptied of DNA in a ping–pause–pong experiment. The brightness and contrast settings of the images incanddwere identical. Images were recorded every 10 s with a 50-ms exposure time. To ensure the incubation times in YOYO-1 were the same, bothcanddare the 50th frames of their respective videos, which correspond to a moment 10 min after the start of the fluorescence measurement. The spot incremained bright for all 154 frames, indicating the cage trapped the DNA for over 25 min. Scale bars, 10 μm. NA, numerical apperture. Figure 7d shows the results of a control experiment where we used the ping–pause–pong procedure to pull the DNA molecule into the cavity, pause for 5 s and then remove it before transferring the device to the microscope. As expected, no flourescence was visible since no molecule was in the cage. The result of this control experiment was reproduced on a second nanopore device. Figure 7: Imaging a trapped DNA molecule. ( a ) Schematic showing one drop of solution containing YOYO-1 fluorescent dye added to the opening side of a chip on an optical microscope. ( b ) An image of a device with a trapped DNA molecule illuminated by white light. The bright square is the three-layer membrane. The disk indicated by a white dashed circle is the cavity. ( c ) A fluorescence image of the same device as in b . ( d ) A fluorescence image of a cage that was emptied of DNA in a ping–pause–pong experiment. The brightness and contrast settings of the images in c and d were identical. Images were recorded every 10 s with a 50-ms exposure time. To ensure the incubation times in YOYO-1 were the same, both c and d are the 50th frames of their respective videos, which correspond to a moment 10 min after the start of the fluorescence measurement. The spot in c remained bright for all 154 frames, indicating the cage trapped the DNA for over 25 min. Scale bars, 10 μm. NA, numerical apperture. Full size image Cutting trapped DNA molecules with a restriction endonuclease We used an entropic cage to subject trapped DNA molecules to a sequence-specific biochemical reaction, as illustrated in Fig. 8a . Buffer containing the SmaI restriction endonuclease was added to the reservoir on the opening side, while the reservoir on the nanopore side was filled with a similar buffer that contained λ DNA instead of the enzyme. We used the ping–pause–pong technique to draw a DNA molecule into the cage, where it could interact with SmaI during the pause, and then reverse the voltage so that the nanopore would interrogate the products of the reaction. SmaI cuts double-stranded DNA at a particular recognition sequence found at three sites along λ DNA. We therefore expected a λ DNA molecule entering the cage to be cut into as many as four pieces, with the number of pieces increasing as the reaction progresses to completion. 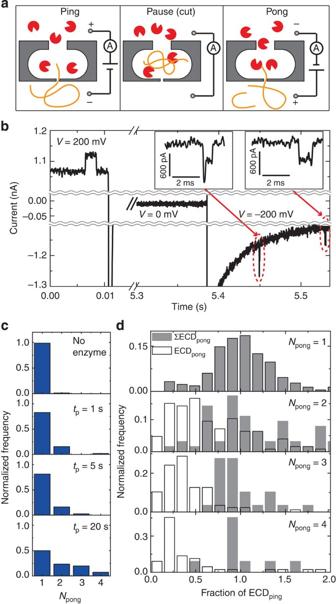Figure 8: Enzymatic cutting of trapped DNA. (a) Illustration of the experiment. (b) A typical current trace showing a single ping followed by two pongs after a pause oftp=5 s. The ECD of the ping is 0.10 pC and those of the pongs are 0.05 and 0.04 pC, sequentially. The wavy lines indicate breaks in the current axis. The current transients near 0.01 and 5.4 s were caused by sudden changes inV. (c) Distributions of pongs per ping–pause–pong cycle,Npong, for three differenttpwith SmaI present, and fortp=5 s without SmaI. The number of ping–pause–pong cycles performed was 62 withtp=1 s, 93 withtp=5 s, 82 withtp=20 s and 76 with no enzyme present. (d) Distributions of(white bars) and(grey bars). Both distributions are normalized by the total number of counts, respectively. Figure 8: Enzymatic cutting of trapped DNA. ( a ) Illustration of the experiment. ( b ) A typical current trace showing a single ping followed by two pongs after a pause of t p =5 s. The ECD of the ping is 0.10 pC and those of the pongs are 0.05 and 0.04 pC, sequentially. The wavy lines indicate breaks in the current axis. The current transients near 0.01 and 5.4 s were caused by sudden changes in V . ( c ) Distributions of pongs per ping–pause–pong cycle, N pong , for three different t p with SmaI present, and for t p =5 s without SmaI. The number of ping–pause–pong cycles performed was 62 with t p =1 s, 93 with t p =5 s, 82 with t p =20 s and 76 with no enzyme present. ( d ) Distributions of (white bars) and (grey bars). Both distributions are normalized by the total number of counts, respectively. Full size image Figure 8b shows a typical current trace obtained with t p =5 s. Applying V =200 mV drew a DNA molecule into the cage through the nanopore, in this case causing an increase in I because the DNA is highly charged and therefore entrains enough counterions into the nanopore to increase its conductance in low-salinity enzyme buffer [40] . After the pause, the voltage was flipped to V =−200 mV and maintained for 5 s. From the single ping, we obtained two pong signals in this case, indicating that a molecule was trapped inside the cavity, cut and pulled back through in pieces. We varied t p in our experiments between t p =1, 5 and 20 s to probe the restriction reaction after different incubation times. At each t p , we repeated the experiment at least 60 times. We also performed control experiments with no SmaI present and t p =5 s. Figure 8c shows the distribution of the number of pongs observed per ping–pause–pong cycle ( N pong ) for the different incubation times and for the experiment with no enzyme. Between one and four molecules were recaptured per cycle. Without SmaI, 98.6% of the experimental cycles returned only one pong. With SmaI present, the probability of detecting multiple pongs in a cycle increased with t p , from 17.3% at t p =1 s to 50.0% at t p =20 s. To confirm that multiple pong signals were caused by fragments of the original molecule, we verified that the fragments were smaller than the original molecule and compared the total size of the recaptured fragments in a cycle with the size of the original molecule, using ECD as a measure of size. Figure 8d shows the distributions of , the ECD values of the pongs relative to the corresponding ping, grouped by N pong (white bars). That figure also plots the distributions of , the total ECD of all the pongs in a cycle relative to the corresponding ping (grey bars). When N pong =1, the distribution of was centred around 1, indicating that the molecule was not cut because its size did not change. As more pongs were detected per cycle, the distribution of shifted to lower values, indicating that the recaptured molecules were becoming smaller than the original one. The peak of the distribution remained near 1 for all N pong , however, indicating that the total size of the recaptured molecules was the same as the original. Finally, Fig. 9 is a scatter plot of pong events from the enzymatic cutting experiments indicating t r and ECD. Molecules that had not been cut gave pongs in the high ECD, short t r region of the data, while the fragments produced by the restriction digest gave pongs in the low ECD, long t r region. These results reflect the fact that short DNA fragments, which give low ECD, have a relatively high diffusivity [31] , so they can more easily diffuse away from the nanopore. We note that these results are also consistent with Grosberg’s model of the DNA capture rate in the regime, where the rate is limited by an entropic barrier [38] ; within that model, the low effective charge of short polymer fragments can more easily resist the weakened pull of the electrophoretic force. Fragments consequently exhibited longer recapture times than intact λ DNA molecules. This also explains the data in Fig. 4a,b , which show that short DNA fragments, as measured by ECD, resulted in the longest t r . 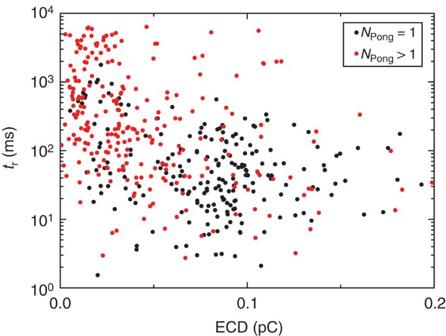Figure 9: Scatter plot of pong events from the enzymatic cutting experiments indicatingtrand ECD. Cycles withNpong=1 gave the intact molecules indicated in black. Cycles withNpong>1 yielded the fragments indicated in red. These enzymatic cutting experiments used a low-salinity buffer solution that gave lower ECD values for intact λDNA molecules than in other ping–pause–pong experiments performed using a high-salinity solution. Figure 9: Scatter plot of pong events from the enzymatic cutting experiments indicating t r and ECD. Cycles with N pong =1 gave the intact molecules indicated in black. Cycles with N pong >1 yielded the fragments indicated in red. These enzymatic cutting experiments used a low-salinity buffer solution that gave lower ECD values for intact λDNA molecules than in other ping–pause–pong experiments performed using a high-salinity solution. Full size image We have demonstrated that entropic cages can capture single DNA molecules next to a nanopore. We have confirmed this by observing plateauing recapture time and high recapture probability in devices with cages, and by directly imaging trapped molecules using fluorescence microscopy. The ability to capture and constrain a single molecule allows us to study the physics of a molecule’s translocation of a nanopore in general, since it affords us some control over the state of the molecule before reverse translocation [7] , [41] , [42] , [43] . Entropic traps also enhance solid-state nanopore technology by serving as single-molecule test tubes in which a molecule, interrogated by the nanopore on the way in, can react and then be probed again on the way out. As an example, we demonstrated the cutting of a trapped DNA molecule in the cavity, which can provide a way to simulate the restriction modification systems of bacteriophage resistance mechanisms [44] in vitro . In addition, compared with the widely used genomic analysis method of optical mapping [45] , [46] , [47] , which uses a microscope to observe the results of cutting long, single DNA molecules with restriction enzymes, our device provided a fast and label-free way to study the enzymatic cutting of DNA in real time. Given careful choice of enzyme and more thorough study of the reaction conditions, one could use the device to study genetic variations using restriction fragment length polymorphisms [48] . Nanopore devices Silicon chips with freestanding membranes suspended over 50-μm-wide square openings were microfabricated by standard procedures described in detail elsewhere [49] . We fabricated nanopore cage structures following the procedure described in the nanopore cage structure and experiments subsection of the Results. Prior to a DNA-sensing experiment, each device was cleaned in Nanostrip (Cytantek corporation) at 75 °C for 2 h, and its ionic conductance was tested in the presence of 1 M KCl buffer to ensure that the s.d. of the baseline current in a 1-min recording was no greater than 0.01 nA with V =100 mV. Chemicals and buffers The buffer used to study recapture times in ping–pause–pong experiments contained 1 M KCl, 10 m M Tris and 1 m M EDTA at pH=8. 1. Twenty-five μg ml −1 λ DNA (New England Biolab, N3011S) was added to the buffer in the nanopore reservoir. To stain trapped DNA for fluorescence optical microscopy, we used a 5-μ M solution of YOYO-1 dye (Invitrogen) in 20 m M Tris-HCl, 1 m M EDTA at pH 8.0. The buffer used to perform the enzymatic DNA-cutting experiment contained 50 m M potassium acetate, 20 m M tris-acetate, 10 m M magnesium acetate, 1 m M dithiothreitol, at pH=7.9, where the SmaI restriction endonuclease (New England Biolab, R0141S) is active at room temperature (24 °C). We added 1.25 μg ml −1 λ DNA to the nanopore side and 400 units per ml SmaI enzyme (~14 nM) to the opening side. All buffer solutions used in DNA-sensing experiments were degassed under vacuum for 1 h before use. The DNA suspensions were heated to 65 °C for 10 min and then quickly cooled to room temperature to separate the complementary overhanging ends of λ DNA and thereby avoid concatenated or circular molecules. Electrical control and signal processing I was monitored by an electrometer (Axon Axopatch 200B), whose output was conditioned by an analogue, eight-pole, low-pass Bessel filter with a 10-kHz cutoff (Stanford Research Systems), and digitally sampled at 250 kHz. The filtered output of the current amplifier was simultaneously monitored by a FPGA (NI PCI-7830R) running a custom LabView program, which executed ping–pause–pong cycles. The FPGA controlled V by means of an analogue voltage command line to the electrometer. A ping–pause–pong cycle was triggered in experiments performed in 1 M KCl solution by a decrease in the current from the baseline that exceeded 0.1 nA and that lasted longer than 200 μs. In the enzymatic DNA-cutting experiments, which were performed in a lower ionic strength solution, a ping–pause–pong cycle was triggered by an enhancement of the current above the baseline of 0.04 nA or more and lasting 100 μs or longer. Experimental controls We ensured that our measurements of t r and the recapture probability were not confounded by molecules that were left over on the opening side of the device from an earlier ping–pause–pong cycle, where, for example, a captured molecule failed to trigger a ping or was not recaptured within the 5 s allotted. Between sets of experiment with different t p , we checked that the opening side was clean by applying V =−100 mV for 1 min. We usually detected no translocations during this time. Only in a few experiments was a single event observed during 1 min, which indicated that molecules left over from previous ping–pause–pong cycles had negligible influence on subsequent experiments. Similarly, we confirmed that the multiple pongs observed in the enzymatic DNA-cutting experiments were not caused by enzyme molecules translocating the nanopore. We applied V =−200 mV for 1 min between sets of experiments using a different t p . No translocation signals were detected, which indicated the SmaI molecule is too large to translocate the nanopore or its translocation signal is too short to be detected. Fluorescence imaging After a DNA-trapping experiment, we removed the nanopore chip from its fluidic chuck, rinsed it in distilled, deionized water to wash away any DNA stuck to the membrane, placed the chip on a microscope cover glass with the opening side facing up, added a small drop of YOYO-1 solution to the opening side and then placed another cover glass on top to prevent evaporation. We mounted the chip sandwiched between cover glasses on an inverted microscope (Nikon, ECLIPSE TE2000-U) equipped with a × 100, oil-immersion objective lens (Nikon, CFI Apo TIRF), an ultraviolet light source (EXFO X-Cite 120), a fluorescence imaging filter set (C125492, Chroma Technology Corp.) and an EMCCD camera (Andor, iXon). Fluorescence images were recorded every 10 s using a 50-ms exposure time and a mechanical shutter that minimized photobleaching. Baseline subtraction from pong events We fit and subtracted the baseline beneath pong events when that baseline was recovering from a sudden change in voltage, as can be seen in Figs 2b , 3a,b and 8b . We fit a 4th-order polynomial to a section of I ( t ) containing the pong event using an asymmetric Huber cost function [50] . Specifically, the best fit, 4th-order polynomial, f ( t ), is the one that minimizes the cost function where is the asymmetric Huber function We used the threshold s =10 pA. increases slowly when x > s , which limits the influence of the pong event on the fit to the baseline. The MatLab software we used is available online at ( http://www.mathworks.com/matlabcentral/fileexchange/27429-background-correction ). How to cite this article: Liu, X. et al . Entropic cages for trapping DNA near a nanopore. Nat. Commun. 6:6222 doi: 10.1038/ncomms7222 (2015).